Reply to: No specific relationship between hypnotic suggestibility and the rubber hand illusion 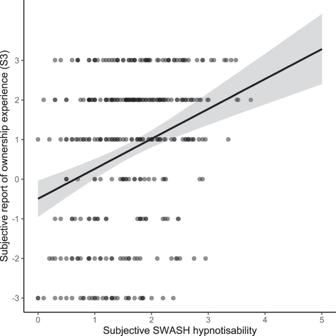Fig. 1: Agreement with the statement “I felt as if the rubber hand were my hand” (S3; ‘ownership’) on hypnotisability. b= 0.76 Likert units subjective response per SWASH unit,SE= 0.13,t= 5.79,P< 0.001, 95% CI [0.50, 1.01] BH(0,1.4)= 4.2 × 106(B calculated as in Lush et al1.).rs= 0.27, 95% CI [0.17, 0.36]. Source data are provided as a Source Data file. Further information on research design is available in the Nature Research Reporting Summary linked to this article.